Radical SAM-dependent ether crosslink in daropeptide biosynthesis Darobactin is a ribosomally synthesized and post-translationally modified peptide (RiPP), which possesses potent activity against various Gram-negative bacteria. Darobactin features a highly unique bicyclic scaffold, consisting of an ether crosslink between two Trp residues and a C–C crosslink between a Lys and a Trp. Here we report in vivo and in vitro activity of darobactin synthase DarE. We show DarE is a radical S-adenosylmethionine (rSAM) enzyme and is solely responsible for forming the bicyclic scaffold of darobactin. DarE mainly produced the ether-crosslinked product in vitro, and when the assay was performed in H 2 18 O, apparent 18 O incorporation was observed into the ether-crosslinked product. These observations suggested an rSAM-dependent process in darobactin biosynthesis, involving a highly unusual oxygen insertion step from a water molecule and subsequent O–H and C–H activations. Genome mining analysis demonstrates the diversity of darobactin-like biosynthetic gene clusters, a subclade of which likely encode monocyclic products with only an ether linkage. We propose the name daropeptide for this growing family of ether-containing RiPPs produced by DarE enzymes. The emergence of antimicrobial resistance is one of the major threats to global public health. This situation is especially troublesome with respect to pathogenic Gram-negative species, such as Acinetobacter baumannii , Klebsiella pneumoniae , Pseudomonas aeruginosa and Enterobacter spp . These Gram-negative bacteria are intrinsically resistant to many antibiotics, largely because of the low-permeability barrier resulting from the densely packed lipopolysaccharides in outer membrane [1] . Discovery of novel antibiotics to act against Gram-negative bacteria is challenging, and most frontline antibiotics (e.g., aminoglycosides, tetracyclines, β-lactams, fluoroquinolones) were introduced half a century ago. Due to the increased knowledge of bacterial genomes and the biosynthetic gene clusters (BGCs) of natural products, mining untapped groups of bacteria could perhaps be a fruitful strategy in finding antibiotics with novel scaffolds and modes of action [2] , [3] . Darobactin is a heptapeptide antibiotic found by an activity-based screening effort on nematophilic bacteria [4] . Darobactin features a unique bicyclic scaffold, comprising an ether linkage (C–O–C) between the C7 of W 1 and the C β of W 3 , and a C–C crosslink between the C6 of W 3 and the C β of K 5 (Fig. 1a ). Darobactin targets the bacterial insertase BamA, a central unit of the β-barrel assembly machinery (BAM) complex that is essential for the folding and insertion of outer membrane proteins [5] . The bicyclic scaffold of darobactin adopts a rigid β-strand conformation, thereby allowing the molecule to bind the lateral gate of BamA with an affinity in submicromolar range [6] . Darobactin exhibits potent activity against various multi-drug resistant Gram-negative bacteria both in vitro and in animal models. Moreover, it shows no activity against common symbiotic gut bacteria and human cell lines, presenting as a promising lead compound for developing therapeutics against Gram-negative pathogens [4] . Fig. 1: Darobactin and its BGC. a The chemical structure of darobactin. The key C–O–C and C–C crosslinks that consist the unique bicyclic scaffold of darobactin are highlighted in blue. b The darobactin BGC from Photorhabdus khanii HGB1456 encodes a precursor peptide DarA pk , an rSAM enzyme DarE pk , and three ABC transports DarBCD pk . The core sequence of DarA pk (DarA pk(49-55) ) is shown in bold. Full size image Darobactin belongs to the ribosomally synthesized and post-translationally modified peptide (RiPP) superfamily [7] , [8] . The darobactin BGC encodes a 58-amino acid (aa) precursor peptide DarA, a radical S-adenosylmethionine (rSAM) enzyme DarE, and an ABC-type transporter DarBCD (DarB and DarD are the transporters whereas DarC is a membrane fusion protein) (Fig. 1b ) [4] . The rSAM superfamily enzymes are extensively involved in RiPP biosynthesis and catalyze strikingly diverse reactions [9] , [10] , [11] . The rSAM-dependent cyclic RiPPs include sactipeptide (α-thioether linkage) [12] , [13] , [14] , [15] , [16] , [17] , [18] , ranthipeptide (β or γ-thioether linkage) [19] , [20] , [21] , lytreptides (C–C crosslink between Lys and Trp) [22] , [23] , rotapeptide (C–O crosslink between Thr and Gln) [24] , ryptide (C–C crosslink between Arg and Tyr) [25] , triceptide (C–C crosslink between an aromatic aa and a non-aromatic aa) [26] , [27] , among others (Supplementary Fig. 1 ). However, the bicyclic scaffold of darobactin, particularly the ether crosslink between two Trp residues, is distinct from all the known rSAM-dependent RiPPs. Recent heterologous expression studies showed that the minimum darobactin BGC consists of only darA and darE , whereas darBCD is not essential for darobactin production [27] , [28] , [29] . However, the pathway for darobactin maturation and the exact function of DarE remains unclear. Herein, we show DarE is solely responsible for the bicyclic scaffold formation in darobactin biosynthesis. We also show darobactin analogs are widespread in nature with high structural diversity, and we propose the name daropeptide for this growing family of RiPPs. In vivo activity of DarE pk To investigate darobactin biosynthesis, we coexpressed darE from Photorhabdus khanii HGB1456 with its precursor peptide gene darA in Escherichia coli (the two genes are referred to as darE pk and darA pk to differentiate from the homologs from other strains). In contrast to the recent coexpression studies that focused on darobactin production [28] , [29] , we expressed darA pk with an N-terminal hexa-histidine tag (Supplementary Fig. 2 ) and purified the peptide by Ni 2+ -affinity chromatography. Liquid chromatography with high-resolution mass spectrometry (LC-HRMS) analysis showed the resulting DarA pk exhibited a protonated molecular ion at [M + 8H] 8+ = 1011.0, which is 12 Da higher than the expected unmodified DarA (hereafter the fully modified +12 Da peptide is termed DarA pk - 1 ) (Fig. 2a ). DarA pk - 1 was then digested by trypsin and analyzed by high-resolution MS (HR-MS) (Fig. 2a ) and tandem MS (HR-MS/MS) (Supplementary Fig. 3 ). This analysis clearly revealed that the tryptic fragment DarA pk(43-58) -1 ([M + 2H] 2+ cal. 980.9756, obs. 980.9756, err < 0.1 ppm) contains the expected crosslink between Trp49 and Lys53 (Fig. 1a ), suggesting that the DarE enzyme is responsible for installing the characteristic bicyclic scaffold of darobactin on DarA. Further introduction of darBCD pk into the coexpression system (to avoid any possible issues in relation to gene regulation, all the genes were each expressed under the control of a separate T7-lac promoter, Supplementary Fig. 2 ) did not have an observable effect in the yield and modification pattern of DarA pk (Supplementary Fig. 4 ). This observation suggests that DarBCD do not play an essential role in darobactin biosynthesis, which is consistent with the recent heterologous studies [28] , [29] , [30] . Fig. 2: LC-HRMS analysis of DarA pk produced in vivo, showing the extracted ion chromatograms (EICs) and MS spectra. a DarA pk produced by coexpression with DarE pk carries a + 12 Da modification. Because heterologous expression in E. coli only produced obtained the truncated DarA pk , the theoretically predicted signals corresponding to the unmodified DarA pk were shown for comparison. See Supplementary Fig. 3 for the HR-MS/MS spectrum of DarA pk(43-58) - 1 . b DarA pk produced by coexpression with the C86A mutant of DarE pk is a truncated peptide (i.e., DarA pk(1-48) ), which lacks the core and follower regions. Full size image The rSAM superfamily enzymes utilize a [4Fe-4S] cluster to reductively cleave S-adenosylmethionine (SAM) to generate an extremely reactive 5'-deoxyadenosyl (dAdo) radical, which initiate highly diverse reactions [31] , [32] . This [4Fe-4S] cluster is bound by three Cys residues, which are usually organized in a CxxxCxxC motif. In our analysis, we changed Cys83 in the CxxxCxxC motif of DarE pk (i.e., CNLRCTYC) to an Ala, and the mutant gene was coexpressed with darA pk , using the same protocol as that for the wild type darE pk . Subsequent LC-HRMS analysis showed that the expected unmodified DarA pk was not observed in the purified peptide sample. Instead, the resulting peptide is a truncated peptide DarA pk(1-48) that only contains the leader region of DarA pk , whereas the core and follower peptide regions (i.e., W 49 NWSKSFQEI 58 ) were removed from the precursor peptide (Fig. 2b ). This observation suggests that the leader peptide of DarA pk is naturally cleaved by one or more unknown hydrolases in the proteome of E. coli (as well as the native host P. khanii ). Formation of the bicyclic scaffold of darobactin likely decreases the proteolysis efficiency, allowing for the purification of the full-length modified DarA pk -1 in our analysis (Fig. 2a ). Similar to the recent reports [28] , [29] , production of the mature darobactin is also observed in our analysis (Supplementary Fig. 5 ). To show that cleavage of DarA leader and follower peptide was achieved by E. coli proteins, we incubated the in vivo modified DarA pk - 1 with the cell lysate of E. coli BL21. In this analysis, we saw apparent production of darobactin in the reaction (Supplementary Fig. 6 ). This result clearly demonstrates that proteolytic cleavage of DarA for darobactin maturation is catalyzed by one or more unknown hydrolases in the E. coli proteome. In vitro analysis of DarE pk We next set out to investigate the in vitro activity of DarE pk . To this end, we overexpressed DarE pk in E. coli with an N-terminal hexa-histidine tag. However, despite extensive efforts the protein was mainly seen in the inclusion bodies. Because in our coexpression study DarE pk is apparently functional and can efficiently install the bicyclic scaffold on DarA pk , we reasoned the presence of the precursor peptide could likely assist the folding of DarE pk . Indeed, coexpression of the untagged DarA pk with the N-terminally His-tagged DarE pk significantly increased protein solubility. By this approach ~30 mg DarE pk was obtained from 2 L cell culture by Ni 2+ -affinity chromatography under strictly anaerobic conditions. The as-isolated protein appeared brownish and exhibited a weak broad absorption around 410 nm, and this absorption band significantly increased after chemical reconstitution of the [4Fe-4S] cluster (Supplementary Fig. 7 ). Quantification analysis showed that each enzyme contains 7.8 ± 0.5 iron and 7.2 ± 0.6 labile sulfide, suggesting it harbors two [4Fe-4S] clusters. This observation is consistent with the fact that DarE contains a C-terminal SPASM/twitch domain, which binds additional [4Fe-4S] clusters, with roles suggestive of peptide binding or electron transfer [33] , [34] . Anaerobic incubation of the reconstituted DarE pk with SAM and sodium dithionite (DTH) produced a significant amount of 5ˊ-deoxyadenosine (dAdoH) (Supplementary Fig. 7 ), validating that DarE pk is an rSAM enzyme. Similar to the above-mentioned efforts in coexpression of DarA pk with the C83A mutant of DarE pk , expression of DarA pk alone in E. coli only afford the truncated peptide DarA pk(1-48) . We hence obtained the full-length DarA pk by solid-phase peptide synthesis (SPPS) (Supporting Methods), and the assay was then performed by treating DarA pk with the reconstituted DarE pk , SAM, and DTH under strictly anaerobic condition. The reaction mixture was then treated with trypsin and analyzed by LC-HRMS. This analysis revealed an apparent product corresponding to the tryptic fragment DarA pk(43-53) (i.e., I 43 PEITAWNWSK 53 ) harboring +14 Da modification ([M + 2H] 2+ cal. 679.8406, obs. 679.8505, err. 0.1 ppm), and this product was clearly absent in the control assays with the supernatant of boiled enzyme (Fig. 3a ). The +14 Da tryptic product (hereafter referred to as DarA pk(43-53) - 2 ) is consistent with the modified DarA pk containing an ether crosslink between Trp49 and Trp51, which is further supported by HR-MSMS analysis (Supplementary Fig. 8 ). Fig. 3: In vitro analysis of DarE pk . a The EIC and HRMS spectrum corresponding to the tryptic fragment DarA pk(43-53) - 2 , which contains an ether-crosslink between Trp49 and Trp51. b The EIC and HRMS spectrum corresponding to the tryptic fragment DarA pk(43-53) - 1 containing the fully modified bicyclic scaffold. c The EIC and HRMS spectrum corresponding to the tryptic fragment DarA pk(43-53) - 3 likely containing a dehydrogenated Trp51 (dhW). Trace i, ii, and iii correspond to the full reaction, the solution of reconstituted DarE pk , and the negative control with the supernatant of heat-inactived enzyme. d HRMS spectra of the tryptic fragments DarA pk(43-53) - 2 generated in (i) a buffer containing ~80% H 2 18 O, which was obtained by ultrafiltration and H 2 18 O dilution. The asterisk indicates 18 O incorporation (~50% enrichment) into the resulting peptide. A control experiment (ii) was performed in parallel with H 2 O. See Supplementary Fig. 12 for the detailed comparison of the HR-MSMS spectra for the 18 O-labeled vs. unlabeled tryptic fragments DarA pk(43–53) − 2 . Full size image We also observed a trace amount of fully modified DarA pk harboring the +12 Da modification (i.e., DarA pk - 1 ), whose tryptic fragment DarA pk(43-58) - 1 exhibit a protonated molecular ion at [M + 2H] 2+ = 980.9756 (cal. 980.9756, err. <0.1 ppm) (Fig. 3b ). Although the in vitro reaction efficiency of DarE pk is low and needs further optimization, these results clearly demonstrate that DarE installs the bicyclic scaffold of darobactin on DarA via rSAM-dependent chemistry. We did not observe the product corresponding to the peptide only containing the Trp51-Lys53 crosslink (i.e., having a C–C crosslink but lacking the ether linkage). Together with the fact that the ether-crosslinked DarA pk - 2 is the major product in the assay, this observation suggests that ether bond formation between Trp49 and Trp51 is likely the first step in darobactin biosynthesis. We also constructed a K53A mutant of DarA pk in which the to-be-cyclized Lys53 was changed to Ala, and the mutant was coxpressed with DarE pk . LC-HRMS and HR-MSMS analysis clearly indicated the resulting DarA pk mutant mainly harbored a + 14 modication, which occurred between Trp48 and Trp51 (Supplementary Fig. 9 ). This result is consistent with the proposal that ether bond formation precedes the C–C bond formation in darobactin biosynthesis. Interestingly, careful analysis of the in vitro reaction mixture revealed a tryptic fragment DarA pk(43-53) harboring -2 Da modification ([M + 2H] 2+ cal. 671.8431, obs. 671.8425, err. 0.9 ppm), and this product (hereafter referred to as DarA pk(43-53) - 3 ) was clearly absent in the control assays with the supernatant of boiled enzyme (Fig. 3c ). This −2 Da product is apparently not related to the Trp51-Lys53 crosslink (i.e., the C–C crosslink between W 3 and K 5 in darobactin), which would preclude tryptic cleavage between Lys53 and Ser54. Detailed HR-MS/MS analysis showed the −2 Da modification occurred on Trp51 (Supplementary Fig. 10 ), suggesting the production of dehydrogenated Trp (dhW) in DarE reaction. Dehydrogenation of Trp51 raises an interesting possibility that the β-hydroxyl moiety of Trp in darobactin is likely a result dhW hydration. To test this hypothesis, we performed the assay in a buffer containing ~80% H 2 18 O, and the reaction mixture was examined by HR-LCMS. This analysis clearly revealed 18 O incorporation into the corresponding DarA pk(43-53) - 2 fragment (Fig. 3d ). Detailed HR-MSMS analysis showed that the 18 O atom is incorporated between Trp49 and Trp51 (Supplementary Figs. 11 – 12 ), suggesting the oxygen atom in the ether crosslink of darobactin is derived from H 2 O. Based on the results presented above, we proposed a working hypothesis for the DarE-catalyzed reaction (Fig. 4 ). In the reaction, the dAdo radical generated from SAM cleavage abstracts a hydrogen from the side chain of Trp51, leading to the production of the dhW-containing product DarA- 3 . Because DarE shares apparent sequence similarity with tricepeptide synthases (e.g., 38% similarity with SjiB [27] ), this hydrogen abstraction process very likely occurs on the β-carbon of Trp51 (Fig. 4 ). DarA- 3 is subsequently hydrated via a stereoselective Michael addition to produce DarA- 4 . The dAdo radical produced from the second SAM molecules then abstracts the hydrogen from the β-hydroxyl group of DarA- 4 to produce an oxygen-centered radical X , which then attacks the C7 indole ring of Trp49 to install the C–O–C linkage (Fig. 4 ), in a way similar to that proposed in glycopeptide biosynthesis [35] , [36] . It is noteworthy that although hydrogen abstraction from an alcohol hydroxyl group is rare in biochemistry, this type of chemistry has been demonstrated in NosL catalysis with unnatural substrates [37] , [38] , [39] . After the formation of the ether crosslink, the dAdo radical from the third SAM molecule then installs the C–C crosslink between Lys53 and Trp49; similar type of chemistry has been well characterized in various rSAM-dependent RiPPs such as streptide [22] , [23] . Owing to the complex chemistry of DarE, further investigations are awaited to validate the detailed mechanism of this remarkable catalytic process. Fig. 4: A proposed mechanism for the DarE-catalyzed bicyclic crosslinking. N in the circle represents the Asn residue between the two Trp residues in DarA (e.g., N 2 in darobactin). Full size image The substrate diversity of DarE enzymes Recent heterologous studies demonstrated the great potential to expand the structural diversity of daropeptide by bio-engineering efforts [28] , [29] . To explore the catalytic protential and substrate specificity of DarE enzymes, we carried out a BLASTp search in UniProt database using DarE pk as query sequence. The putative darobactin synthases were then selected by analyzing the neighboring sequences of these enzymes with the assistance of the EFI-genome neighborhood tool [40] . The identified enzymes were then incorporated into a sequence similarity network (Fig. 5a ), and the corresponding precursor peptides were analyzed by multiple sequence alignment (Fig. 5b ). Fig. 5: Diversity and classification of darobactin-like BGCs. a The sequence similarity network of DarE enzymes. Each node in the network represents a putative DarE sequence, and each edge represents sequences with BLASTP E values below 1E-165. b The conserved core sequences in the putative precursor peptides are shown by black bars. Full size image In this analysis, putative DarE enzymes appear to fall into four clusters (Fig. 5a ), and the corresponding precursor peptides in each cluster also contain different core sequences (Fig. 5b ). The cluster I consists of sequences from Photorhabdus , which includes the known darobactin synthase DarE pk . The precursor peptides from cluster I contain the conserved WNWxKxF core peptide, representing the typical bicyclic scaffold of darobactin. Cluster II consists of sequences from diverse genera, and the core peptides WNWSKSF are similar to those from cluster I, but these precursor peptides mostly do not have a follower sequence (e.g., the last two aa in DarA pk ). Cluster III mainly consists of sequences from Yersinia , and the precursor peptides contain a WNWx(K/R)xF core, suggesting the crosslinked Lys could be replaced by an Arg. Like cluster I, the sequences from cluster IV are also from Photorhabdus ; however, the precursor peptide sequences of cluster IV (WT(F/Y)RF) are apparently distinct from those of the other three clusters. To interrogate the DarE-catalyzed modification on other precursor peptides, we first focused on a cluster III BGC from Yersinia intermedia , which encodes a precursor peptide (hereafter DarA yi ) containing an Arg substitution in the core (i.e., WNWS R SF). Similar to the coexpression study discussed above, we coexpressed DarA yi in an N-terminal hexa-histidine tagged form with the corresponding modifying enzyme DarE yi , and the resulting peptide was purified by Ni 2+ -affinity chromatography. LC-HRMS analysis revealed an apparent peak of +12 Da relative to the unmodified DarA yi (Fig. 5a ) consistent with the formation of the expected bicyclic scaffold. Upon trypsin digestion followed by LC-HRMS analysis, we observed a peptide fragment exhibiting a protonated molecular ion at [M + 2H] 2+ = 740.3349 (cal. 740.3362, err. 1.7 ppm), which corresponds to the fully modified C-terminus of DarA yi (i.e., DarA yi(55-66) - 1 ) (Fig. 6a ), and the crosslink between Trp58 and Arg62 is further supported by HR-MS/MS analysis (Supplementary Fig. 13 ). Fig. 6: An Arg-containing daropeptide from Yersinia intermedia . a HRMS analysis of the fully modified DarA yi (DarA yi -1 ) produced by coexpression of DarA yi with DarE yi . Similar to Fig. 1 , the theoretically predicted signals corresponding to the unmodified DarA yi were shown for comparison. b The chemical structure of DarA yi(55-66) -1 , showing the key NOSEY correlation. See Supplementary Figs. 10 – 13 for the 1D and 2D NMR spectra and Supporting methods for details. Full size image To validate that the bicyclic scaffold produced on DarA yi has the same regio- and stereo-chemistry as that of darobactin, we set out to characterize the tryptic fragment DarA yi(55-66) - 1 by NMR. To this end, we performed coexpression experiment in a large scale, and the fully modified DarA yi - 1 was purified from 60 L cell culture and was then treated with trypsin. Multiple rounds of semi-preparative LC, guided by the LC-MS, afford ~1 mg purified DarA yi(55-66) - 1 . 1 H NMR analysis of the resulting compound revealed several exchangeable amide NH protons (δ H 5.6–8.4 ppm), confirming it is a peptide (Supplementary Fig. 14 ). Although a high degree of signal overlap in the 1 H NMR spectrum, twelve spin systems were assembled from the integrative analysis of 2D NMR data, including COSY, HSQC, and NOESY (Fig. 6b , Supplementary Figs. 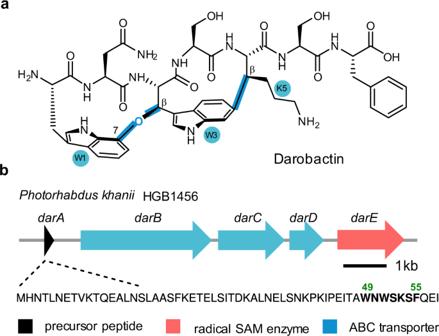Fig. 1: Darobactin and its BGC. aThe chemical structure of darobactin. The key C–O–C and C–C crosslinks that consist the unique bicyclic scaffold of darobactin are highlighted in blue.bThe darobactin BGC fromPhotorhabdus khaniiHGB1456 encodes a precursor peptide DarApk, an rSAM enzyme DarEpk, and three ABC transports DarBCDpk. The core sequence of DarApk(DarApk(49-55)) is shown in bold. 15 – 17 and Supplementary Table 1 ), which are in full agreement with the expected DarA yi(55-66) sequence. Importantly, a significant downfield shift of a doublet at 5.99 ppm (W 4 -Hβ) clearly indicates oxidation of the W4 Cβ, which appear as a methine at 75.19 ppm. By a combination of vicinal coupling ( 3 J), NOESY correlations, and biogenetic considerations, the newly generated two stereocenters at the Cβ of W 6 and R 8 were assigned to be R - and S -configured, respectively. These results revealed the bicyclic scaffold on DarA yi(55-66) is identical to that reported for the darobactins (Fig. 1 ) [4] , [29] . We also performed the density functional theory (DFT) calculation using the gauge-including atomic orbital (GIAO) method [41] , [42] , and the calculation is in good agreement with the experimental data (Supplementary Fig. 18 ). Together, our analysis indicates that DarE installs the characteristic bicyclic scaffold of darobactin on a Lys-to-Arg variant of DarA with the same regio- and stereo-selectivity. We next focused a cluster IV BGC from Photorhabdus asymbiotica (Fig. 6a ). To this end, the precursor peptide DarA pa was coexpressed with the modifying enzyme DarE pa , and the resulting purified peptide was analyzed by LC-HRMS analysis. This analysis showed the resulting DarA pa (i.e., DarA- 1 ) harbors +14 Da modification ([M + 8H] 8+ obs. 929.5505, cal. 929.5506), suggesting the formation of an ether crosslink (Supplementary Fig. 19 ). LC-HRMS analysis of the trypsin-digested sample revealed a peptide fragment (i.e., DarA pa(32-49) -1 ) exhibiting a protonated molecular ion at [M + H] 2+ = 1177.0314 (cal. 1177.0334, err. 1.7 ppm) (Supplementary Fig. 20 ). Subsequent HR-MS/MS analysis clearly revealed the ether crosslink in DarA pa(32-49) -1 is formed between Trp45 and Phe47 (Supplementary Fig. 20 ). This analysis suggested that the class IV BGCs likely encode monocyclic peptides that only contain an ether crosslink. To further test this hypothesis, we performed the in vitro proteolytic assay by treating the in vivo obtained DarA pa - 1 with the cell lysate of E. coli BL21, similar to the in vitro darobactin production discussed above. Indeed, this analysis clearly revealed the production of a compoud exhibiting a protonated molecular ion at [M + H] + = 770.3595 (cal. 770.3620, err. 3.2 ppm) (Figs. 7 b and 7b ). This compound corresponds to a pentapeptide WTFRF containing an ether crosslink between W 1 and F 3 , and this proposal is further supported by HRMS/MS analysis (Supplementary Fig. 21 ). Although we failed to obtain enough amount of peptide for NMR characterization owing to its very low yield, we expect the ether crosslink of DarA pa -1 is formed with the same regio- and stereo-chemistry as that of darobactin. Future studies are awaited to further characterize these monocyclic darobactin-like natural products encoded by the class IV BGCs. Fig. 7: Production of a monocyclic daropeptide from a cluster IV BGC. a The BGC from P. asymbiotic , showing the genes and the precursor peptide sequence, and the core sequence is shown in bold font. Unlike other daropeptide BGCs, this BGC does not encode the DarBCD transporters but encodes a putative N-acetyltransferase. b The EIC at m/z = 770.36 ± 0.01 (corresponding to the monocyclic pentapeptide containing an ether crosslink) of DarA pa - 1 incubated with (i) the cell lysate of E. coli BL21 or (ii) the boiled cell lysate for 24 h. c HR-MS spectrum of the in vitro obtained monocyclic daropeptide. See Supplementary Figs. 17 – 19 for the data in characterization of the DarA pa -derived peptides. Full size image The DarE pa -catalyzed modification on DarA pa suggested that the ether-crosslink can be not only formed between two Trp residues, but also between a Trp and a Phe. To test this hypothesis, we constructed the W51F mutant of DarA pk , in which the following Trp (i.e., W3 in the final product) was changed to a Phe, and the mutant was coexpressed with DarE pk . LC-HRMS and HR-MSMS analysis showed the resulting DarA pk mutant mainly harbored a + 14 Da modication, which occurred between Trp48 and Phe51 (Supplementary Fig. 22 ). This result suggested the ability of ether-crosslink between a preceding Trp and a following Phe is likely common to enzymes from all the clusters. We also constructed the W49F mutant of DarA pk , in which the preceding Trp (i.e., W1 in the final product) was changed to a Phe. LC-HRMS and HR-MSMS analysis showed the resulting DarA pk mutant coexpressed with DarE pk harbored a + 16 Da modification on Trp51, and the ether-crosslink was not formed (Supplementary Fig. 23 ), suggesting that the enzymes appeared unable to form ether-crosslink between a preceding Phe and a following Trp. Observation of the hydroxylated Trp51 in this analysis is also consistent with the mechanisic proposal that W3 is first hydroxylated prior to ether crosslink formation (Fig. 4 ). To test the enzymes of different clusters are promiscuous toward precursor peptides of other clusters, we coexpressed DarA pk with DarE yi and DarE pa , respectively. In contrast to complete formation of the bicyclic strcutre observed for the naitve enzme DarE pk , only ether-crosslink (i.e, +14 Da modification) was observed for the DarA pk peptide coexpressed with DarE yi and DarE pa (Supplementary Figs. 24 – 25 ). These results suggested that although DarA can be modified by DarE enzymes from different clusters, these enzymes are likely not as efficient as the naitve enzyme. Observation of the monocyclic ether-crosslinked DarA pk in these analysis again supported that ether-crosslink precedes the C–C bond formation in darobactin biosynthesis. In summary, we show DarE is solely responsible for producing the bicyclic scaffold of darobactin. This remarkable double crosslinking reaction is dependent on rSAM chemistry, and formation of the ether link between two Trp residues precedes the formation of C–C crosslink of darobactin. Identification of a Trp-dehydrogenated product and isotopic labeling studies shed mechanistic insights into the rSAM-dependent ether crosslinkage, highlighting the remarkable catalytic repertoire and intriguing chemistry of the rSAM superfamily enzymes. Our study also demonstrates a unique RiPP biosynthetic pathway, involving an rSAM-dependent crosslinkage and proteolysis by utilizing the peptidases/hydrolases from the host proteomes. Our study also demonstrates the rich reservoir of darobactin-like BGCs and the potential in investigating this family of RiPPs by genome mining and biosynthetic engineering efforts. Besides the bicyclic scaffold, monocyclic scaffolds with only an ether crosslink can also be produced, which could be the final products (i.e., clade IV BGC) or intermediates resulted from the inefficient enzyme catalysis. We propose the name daropeptides for this growing family of RiPPs that feature an aromatic-aliphatic ether crosslinkage produced by DarE enzymes. Future studies to explore the chemical space and biological activity of this intriguing family of RiPPs could be fruitful, particularly for the development of novel antibiotic lead compounds against Gram-negative pathogens. Production of the DarE-modified DarA The corresponding coexpression plasmids containing both darA and darE genes were transformed into chemical competent BL21(DE3) cells by heat shock. Cells were grown for 16 h on LB agar plate at 37 °C. A single colony transformant was used to inoculate 10 mL of LB medium and grown at 37 °C overnight. This culture was used to inoculate 1 L of TB medium, incubated at 37 °C/200 rpm until an OD 600 of 0.6–0.8 was reached, and then induced with IPTG to a final concentration of 0.2 mM. The cultures were then incubated at 18 °C with for 18 h. The cells were harvested by centrifugation (4000 x g for 10 min), and were directly subjected to protein purification. The cell paste was resuspended in about 20 mL denaturing buffer I (6 M guanidine hydrochloride, 20 mM Tris, 500 mM NaCl, 0.5 mM imidazole, pH = 7.5) and then lysed by sonication on ice. The sample was centrifuged at 12,000 x g for 40 min at 4 °C. The insoluble portion was discarded and the resulting supernatant was clarified through 0.45 mm syringe filters. The peptide-containing sample was the loaded to a 3 ml Ni-NTA column pre-equilibrated with buffer I. The resin was successively washed with 2 column volumes (CV) of buffer I and 4 CV of buffer II (4 M guanidine hydrochloride, 20 mM Tris, 300 mM NaCl, 30 mM imidazole, pH = 7.5), and the desired peptide was eluted using 3 CV of elution buffer (4 M guanidine hydrochloride, 20 mM Tris, 100 mM NaCl, 500 mM imidazole, pH = 7.5). The peptide was then desalted by semi-preparative HPLC using the YMC-Triart C8 column (10.0 × 250 mm, 5 mm). Mobile phase for the crude purification was made of solvent A (0.1% TFA in H 2 O) and solvent B (MeCN). A linear gradient of 5–30% of solvent B over 30 min was executed with a flow rate of 3.0 mL/min. Target peptides were monitored by UV absorbance at 210 and 278 nm, and normally eluted around 20~22 min. Collected fractions were lyophilized and a white fluffy solid was obtained (typically 5 mg of final dried peptide per liter of overexpressed cells), which was further sent for LC-HRMS analysis. LC-HRMS in positive ion mode was operated at 0.3 mL/min with solvent A (0.1% formic acid in H 2 O) and solvent B (MeCN) under the following condition: 0–2 min, 2%B; 2–5.5 min, 2–40%B; 5.5–7.5 min, 40%B; 7.5–9.5 min 95%B. Collision-induced dissociation was a method used for fragmentation, and normalized collision energy was 45 eV. To analyze the proteolysis fragments of the modified substrate DarA, the lyophilized peptides were resuspended in a 100 mL of Tris buffer (20 mM Tris, 25 mM NaCl, pH 8.0) and incubated with trypsin (1:100, trypsin/peptide w/w) at 37 °C for 3 h. After boiling and centrifugation, the supernatant was directly injected to LC-HRMS analysis. The proteolytic digestion of DarA variants using trypsin followed the same procedure unless otherwise specified. In vitro activity assays for DarE pk In vitro assays were usually measured in a 100 µL reaction volume containing DarE (40 µM), precursor peptide DarA (synthesis, 200 µM), sodium dithionite (5 mM), SAM (2 mM) and reaction buffer (50 mM MOPS, pH = 7.5). Boiled enzyme was provided for control assay. The reaction was allowed to process 8–10 h at 30 °C in an anaerobic chamber before quenching with 100 mL MeCN. The precipitant was removed by centrifugation at 13,000 rpm for 15 min and then concentrated volume by SpeedVac for 10 min. 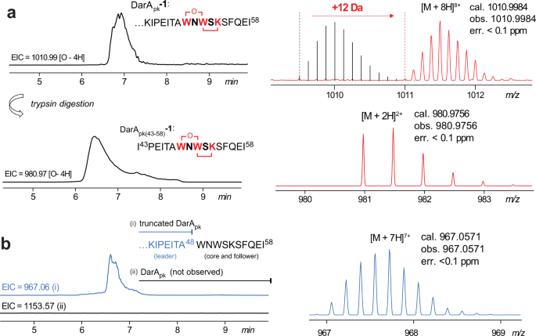Fig. 2: LC-HRMS analysis of DarApkproduced in vivo, showing the extracted ion chromatograms (EICs) and MS spectra. aDarApkproduced by coexpression with DarEpkcarries a + 12 Da modification. Because heterologous expression inE. colionly produced obtained the truncated DarApk, the theoretically predicted signals corresponding to the unmodified DarApkwere shown for comparison. See Supplementary Fig.3for the HR-MS/MS spectrum of DarApk(43-58)-1.bDarApkproduced by coexpression with the C86A mutant of DarEpkis a truncated peptide (i.e., DarApk(1-48)), which lacks the core and follower regions. The supernatant was applied to be analyzed by LC-HRMS. For the assay in H 2 18 O, the reaction mixture was prepared similar to the normal assay with the omitting of SAM. The mixture was then subjected to two rounds of buffer exchange by ultrafiltration and H 2 18 O dilution to achieve a buffer containing ~80% H 2 18 O. The assay was then initiated by addition of the SAM dissolved in H 2 18 O. A parallel experiment performed with ultrafiltration and H 2 O dilution was also performed for comparative analysis. Trypsin digestion of reaction mixture was performed in trypsin digestion buffer (50 mM Tris, 20 mM CaCl 2 , pH = 7.5). 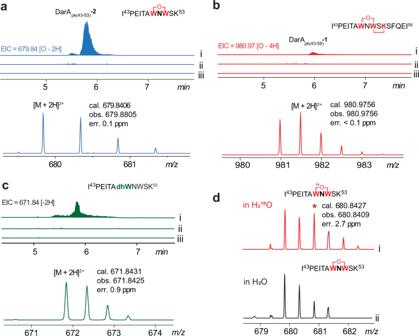Fig. 3: In vitro analysis of DarEpk. aThe EIC and HRMS spectrum corresponding to the tryptic fragment DarApk(43-53)-2, which contains an ether-crosslink between Trp49 and Trp51.bThe EIC and HRMS spectrum corresponding to the tryptic fragment DarApk(43-53)-1containing the fully modified bicyclic scaffold.cThe EIC and HRMS spectrum corresponding to the tryptic fragment DarApk(43-53)-3likely containing a dehydrogenated Trp51 (dhW). Trace i, ii, and iii correspond to the full reaction, the solution of reconstituted DarEpk, and the negative control with the supernatant of heat-inactived enzyme.dHRMS spectra of the tryptic fragments DarApk(43-53)-2generated in (i) a buffer containing ~80% H218O, which was obtained by ultrafiltration and H218O dilution. The asterisk indicates18O incorporation (~50% enrichment) into the resulting peptide. A control experiment (ii) was performed in parallel with H2O. See Supplementary Fig.12for the detailed comparison of the HR-MSMS spectra for the18O-labeled vs. unlabeled tryptic fragments DarApk(43–53)−2. 10 mL freshly prepared trypsin solution (2 mg/ml) was added to 20 mL reaction mixture and replenished the trypsin digestion buffer to a total volume of 50 mL. After incubation at 37 °C for 3 h, 5% (v/v) TFA was added to the solution to quench reaction, and the supernatant was analyzed by LC-HRMS. In vitro proteolysis To prepare the cell lysate, cell pellet of E. coli BL21(DE3) was resuspended in 20 mL of the lysis buffer, lysed by sonication on ice, and centrifugated at 14,000 rpm for 10 mL. 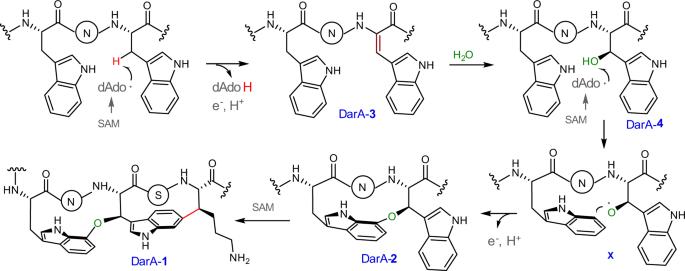Fig. 4: A proposed mechanism for the DarE-catalyzed bicyclic crosslinking. N in the circle represents the Asn residue between the two Trp residues in DarA (e.g., N2in darobactin). 17 mL (1 mg/mL) modified precursor peptide was incubated with 83 mL supernatant of cell lysate. For the control assays, DarA pk -1 was incubated in lysis buffer or treated with the boiled cell lysate. 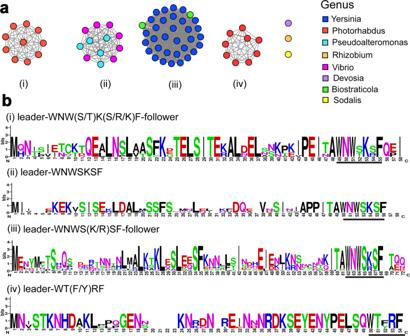Fig. 5: Diversity and classification of darobactin-like BGCs. aThe sequence similarity network of DarE enzymes. Each node in the network represents a putative DarE sequence, and each edge represents sequences with BLASTP E values below 1E-165.bThe conserved core sequences in the putative precursor peptides are shown by black bars. The reaction mixtures were quenched by boiling for 5 min, the precipitated protein was removed by centrifugation, and the respective supernatants were subjected to LC-HRMS analysis. Genome mining To discover DarE homologs, the sequence similarity network (SSN) was constructed by EFI-Enzyme Similarity Tool (EST) [40] ( https://efi.igb.illinois.edu/efi-est/ ) using the Option A ‘sequence BLAST’ with DarE pk (WP_152962147.1) as query input under default parameters (which is used to BLAST in UniProt sequence database to retrieve 5000 sequences with a BLAST E -value at 10 −5 ). The SSN containing 5000 DarE homologs was generated with an E -value cutoff at 10 −170 (90% identical sequences are conflated) and visualized in Cytoscape [43] 3.4.0. using organic layout. The SSN was subsequently uploaded to EFI-genome neighborhood tool (GNT) ( https://efi.igb.illinois.edu/efi-gnt/ ) to manually examine the genomic neighborhood of the 5000 DarE homologs so as to discover BGCs encoding potential darobactin analogs. Multiple sequence alignment of the precursor peptide candidates was generated by using MAFFT. 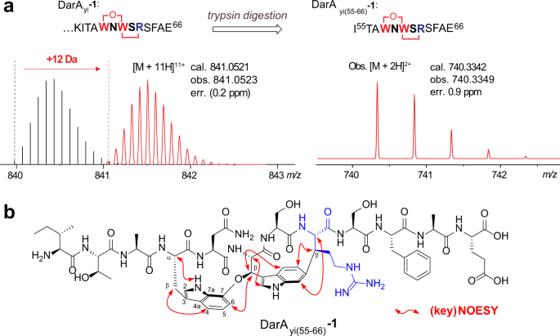Fig. 6: An Arg-containing daropeptide fromYersinia intermedia. aHRMS analysis of the fully modified DarAyi(DarAyi-1) produced by coexpression of DarAyiwith DarEyi. Similar to Fig.1, the theoretically predicted signals corresponding to the unmodified DarAyiwere shown for comparison.bThe chemical structure of DarAyi(55-66)-1, showing the key NOSEY correlation. See Supplementary Figs.10–13for the 1D and 2D NMR spectra and Supporting methods for details. 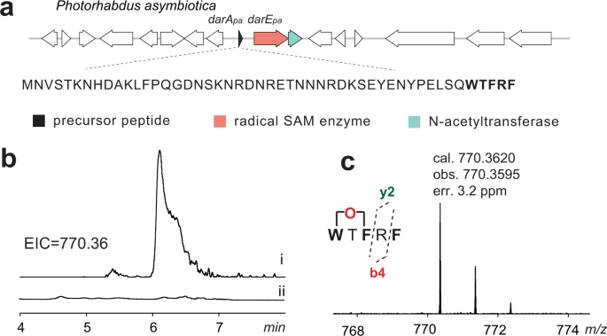Fig. 7: Production of a monocyclic daropeptide from a cluster IV BGC. aThe BGC fromP. asymbiotic, showing the genes and the precursor peptide sequence, and the core sequence is shown in bold font. Unlike other daropeptide BGCs, this BGC does not encode the DarBCD transporters but encodes a putative N-acetyltransferase.bThe EIC atm/z= 770.36 ± 0.01 (corresponding to the monocyclic pentapeptide containing an ether crosslink) of DarApa-1incubated with (i) the cell lysate ofE. coliBL21 or (ii) the boiled cell lysate for 24 h.cHR-MS spectrum of the in vitro obtained monocyclic daropeptide. See Supplementary Figs.17–19for the data in characterization of the DarApa-derived peptides. Sequence logo was generated by using weblogo ( https://weblogo.berkeley.edu/logo.cgi ). Reporting summary Further information on research design is available in the Nature Research Reporting Summary linked to this article.